Respiratory distress and perinatal lethality in Nedd4-2-deficient mice The epithelial sodium channel (ENaC) is essential for sodium homoeostasis in many epithelia. ENaC activity is required for lung fluid clearance in newborn animals and for maintenance of blood volume and blood pressure in adults. In vitro studies show that the ubiquitin ligase Nedd4-2 ubiquitinates ENaC to regulate its cell surface expression. Here we show that knockout of Nedd4-2 in mice leads to increased ENaC expression and activity in embryonic lung. This increased ENaC activity is the likely reason for premature fetal lung fluid clearance in Nedd4-2 −/− animals, resulting in a failure to inflate lungs and perinatal lethality. A small percentage of Nedd4-2 −/− animals survive up to 22 days, and these animals also show increased ENaC expression and develop lethal sterile inflammation of the lung. Thus, we provide critical in vivo evidence that Nedd4-2 is essential for correct regulation of ENaC expression, fetal and postnatal lung function and animal survival. The Nedd4 family of ubiquitin ligases have diverse functions in cellular homoeostasis [1] , [2] , [3] . Nedd4 and its close relative Nedd4-2 ubiquitinate cell surface channels and receptors to promote their internalization and degradation [4] . Nedd4 family members also have roles in other cellular processes, such as endocytosis, viral budding and protein trafficking [4] , [5] , [6] , [7] . In vitro studies suggest Nedd4-2 regulates the heterotrimeric (α+β+γ) amiloride-sensitive epithelial sodium channel (ENaC) [8] , [9] , which is a critical determinant of Na + levels and fluid balance in the body. In the distal nephron, ENaC is essential for Na + resorption to maintain salt homoeostasis, blood volume and blood pressure [10] . In addition, ENaC has a critical role in lung fluid clearance in newborn animals [11] . Mice deficient in the αENaC subunit die within 2 days of birth because of an inability to clear lung fluid, demonstrating the importance of αENaC in this process [11] , whereas the disruption of β or γ subunits has more subtle effects on lung fluid clearance [12] , [13] . In adult lungs, regulation of the amount of luminal fluid on alveolar epithelium is crucial to allow proper gas exchange and alveolar function. The importance of ENaC regulation in adult mice is demonstrated in βENaC transgenic mice, in which the increased expression of βENaC in the lung causes an increase in airway Na + reabsorption resulting in depleted airway surface liquid volume and increased mucous concentration, producing an apparent cystic fibrosis-like lung disease [14] . Nedd4-2 has been shown to regulate ENaC expression at the cell surface [15] . Cytoplasmic PPxY motifs found in all three ENaC subunits interact with WW domains 3 and 4 of Nedd4-2, resulting in downregulation of Na + current due to ubiquitination and subsequent internalization of ENaC [9] , [16] , [17] , [18] . Modulating Nedd4-2 action by glucocorticoids and insulin stimulates ENaC activity [19] , [20] , [21] . Surprisingly, despite the predicted function of Nedd4-2 as a key regulator of ENaC, a Nedd4-2 knockout mouse line generated by Shi and co-workers in a mixed genetic background showed a relatively mild phenotype of salt-sensitive hypertension [22] . We predicted that the genetic background or possible hypomorphic nature of these Nedd4-2 mutant mice may explain the mild phenotype. Here we report on the generation of an independent Nedd4-2 knockout mouse line on a C57BL/6 inbred background. We demonstrate that our knockout represents a null allele of Nedd4-2 and that in the absence of this ubiquitin ligase animals die perinatally with increased ENaC expression and activity in the lung. This leads to a failure to inflate the lungs resulting in an inability of the pups to breathe. Thus, Nedd4-2 is essential for the regulation of ENaC expression in vivo and animal survival. Generation of Nedd4-2 null mice To study the physiological function of Nedd4-2, knockout mice were generated in Bruce4 C57BL/6 embryonic stem (ES) cells to introduce a stop codon in exon 15 of Nedd4-2 ( Fig. 1a ) [23] . We validated that we had created a null allele of Nedd4-2 by immunoblotting E18.5 lung tissue protein lysates that confirmed the absence of Nedd4-2 protein in Nedd4-2 homozygous knockout mice ( Fig. 1b ). Furthermore, we did not detect any Nedd4-2 transcripts in the knockout mice ( Supplementary Fig. S1 ), further validating that our strategy has resulted in a Nedd4-2 null allele (referred to as Nedd4-2 −/− hereafter). Both the Nedd4-2 isoforms present in the Nedd4-2 +/− lung showed approximately half the protein levels of wild-type mice ( Fig. 1b ). The gross morphology of Nedd4-2 −/− pups appeared the same as wild type ( Fig. 1c ). Nedd4 and Nedd4-2 are the two most closely related members of the Nedd4 family and may be able to substitute for each other, but there was no compensatory increase in the expression of Nedd4 observed in the absence of Nedd4-2 ( Fig. 1d ). 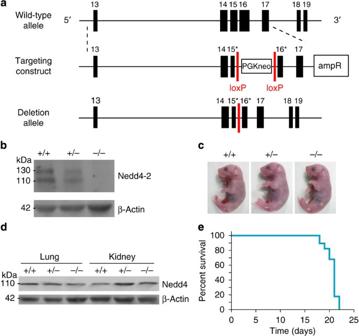Figure 1: Loss ofNedd4-2results in perinatal lethality. (a) Targeting vector design. Top,Nedd4-2wild-type allele exons 13–19 (solid bars). Middle, targeting construct for homologous recombination, with *indicating exonic regions deleted. A stop codon was introduced at exon 15. Bottom, disrupted allele. (b) Nedd4-2 expression in E18.5 lung from wild-type (+/+); heterozygous (+/−) and homozygous (−/−) animals. (c) Gross morphology of E18.5 pups. (d) Nedd4 expression in E18.5 tissues. (e) Survival curve forNedd4-2−/−animals that overcome neonatal death (n=28). Figure 1: Loss of Nedd4-2 results in perinatal lethality. ( a ) Targeting vector design. Top, Nedd4-2 wild-type allele exons 13–19 (solid bars). Middle, targeting construct for homologous recombination, with *indicating exonic regions deleted. A stop codon was introduced at exon 15. Bottom, disrupted allele. ( b ) Nedd4-2 expression in E18.5 lung from wild-type (+/+); heterozygous (+/−) and homozygous (−/−) animals. ( c ) Gross morphology of E18.5 pups. ( d ) Nedd4 expression in E18.5 tissues. ( e ) Survival curve for Nedd4-2 −/− animals that overcome neonatal death ( n =28). Full size image Nedd4-2 −/− animals develop normally but die perinatally The absence of Nedd4-2 −/− pups at the time of weaning (21 days) suggested that the disruption of Nedd4-2 was lethal. Timed matings between Nedd4-2 heterozygotes resulted in embryonic genotypes consistent with Mendelian ratios at both E13.5 and E18.5 ( Table 1 ), suggesting that Nedd4-2 −/− pups die during or shortly after birth. Further observations from more litters revealed that a low percentage ( ∼ 4.2%) of Nedd4-2 −/− animals survived to a maximum of 22 days of age, typically dying at P21 ( Fig. 1e ). Table 1 Survival of Nedd4-2 −/− mice. Full size table To investigate the timing of Nedd4-2 −/− lethality, we performed caesarian recovery on E18.5 embryos. In three litters examined, all Nedd4-2 +/+ and Nedd4-2 +/− pups established rhythmic breathing, a healthy pink skin colour and movement within minutes. However, Nedd4-2 −/− animals turned blue and took short, gasping breaths suggesting these mice could not sufficiently oxygenate their blood. Nedd4-2 −/− pups typically died between 10–60 min after revival, with the exception of a single Nedd4-2 −/− animal that was cyanotic and showed signs of respiratory distress for ∼ 30 min before developing rhythmic breathing and turning pink. We predict that this animal would be one of those ∼ 4.2% animals that lived past birth. A detailed histological analysis of the E18.5 Nedd4-2 −/− mice indicated that they develop normally. All tissues examined including brain, spinal cord, adrenal gland, eye, stomach, small and large intestines, kidney, bone marrow, thymus, spleen, intercostal muscles, heart, skin, liver, bones, pancreas, bladder and testes showed grossly normal morphology (for example, Supplementary Fig. S2 ). Consistent with the respiratory distress phenotype, the only tissue that showed dramatic abnormal morphology was lung, where E18.5 Nedd4-2 −/− animals showed collapsed alveolar spaces and completely failed to inflate the lungs to a functional level ( Supplementary Fig. S2 ). Histological examination of lungs at E15.5 and E17.5 revealed that lung architecture and development was grossly normal in Nedd4-2 −/− animals ( Fig. 2a ). However, at E18.5 the lung architecture was significantly altered in Nedd4-2 −/− animals compared with wild type, with collapsed alveolar spaces resulting in increased tissue density ( Fig. 2a and Supplementary Fig. S2a–d ). To further analyse this phenotype, lungs dissected from Nedd4-2 −/− , Nedd4-2 +/− and Nedd4-2 +/+ caesarian-derived pups at E18.5 were placed in water and observed for flotation to indicate whether respiration had taken place. Whole lungs (including trachea), heart and thymus from Nedd4-2 −/− , Nedd4-2 +/− and Nedd4-2 +/+ floated. However when lungs were dissected into smaller pieces, all individual pieces of Nedd4-2 +/+ and Nedd4-2 +/− lungs floated, whereas approximately half of the individual Nedd4-2 −/− lung pieces sank, indicating that no aeration had occurred in these tissue pieces ( Fig. 2b ). The inability of Nedd4-2 −/− pups to fully aerate their lungs was consistent with their physical signs of respiratory distress. In addition, Nedd4-2 −/− lungs showed a reduced amount of embryonic lung fluid compared with wild type in utero at both E17.5 and E18.5 ( Fig. 2c,d ), presumably leading to the smaller alveolar spaces observed. These observations indicate that loss of Nedd4-2 results in premature lung fluid clearance, leading to a failure to inflate the lungs and subsequent respiratory distress and perinatal lethality. 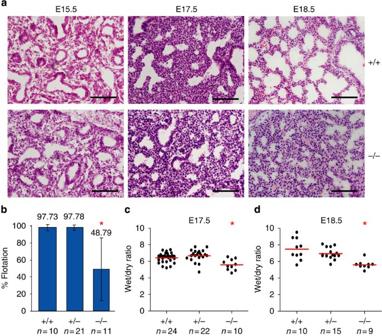Figure 2: Pulmonary abnormalities in embryonic lungs fromNedd4-2−/−mice. (a) Haematoxylin and eosin-stained lung sections. Scale bars, 50 μm. (b) Graphical representation of E18.5 lung flotation rates. Error bars represent the standard deviation. (c) Wet/dry ratio of E17.5 lung tissues. (d) Wet/dry ratio of E18.5 lung tissues. The horizontal lines in red represent the mean value. *For comparison between wild type andNedd4-2−/−standard two-tailed unpairedt-test were performed.P-values are as follows (b)P=0.0005, (c)P=0.0027 and (d)P=0.0004. Figure 2: Pulmonary abnormalities in embryonic lungs from Nedd4-2 −/− mice. ( a ) Haematoxylin and eosin-stained lung sections. Scale bars, 50 μm. ( b ) Graphical representation of E18.5 lung flotation rates. Error bars represent the standard deviation. ( c ) Wet/dry ratio of E17.5 lung tissues. ( d ) Wet/dry ratio of E18.5 lung tissues. The horizontal lines in red represent the mean value. *For comparison between wild type and Nedd4-2 −/− standard two-tailed unpaired t -test were performed. P -values are as follows ( b ) P =0.0005, ( c ) P =0.0027 and ( d ) P =0.0004. Full size image Increased ENaC expression in Nedd4-2 −/− mice At the molecular level, absence of Nedd4-2 is expected to result in decreased ENaC ubiquitination, and therefore less internalization and degradation. To determine whether ENaC expression was altered in Nedd4-2 −/− mice, immunoblot analysis was performed using antibodies generated against α or β subunits of ENaC (specificity of antibodies shown in Supplementary Fig. S3 ). Nedd4-2 −/− E18.5 lung and kidney tissue lysates displayed an increase in α and βENaC expression compared with wild type, with heterozygous mice showing intermediate levels of ENaC expression ( Fig. 3a,b ). Immunostaining of E18.5 lung sections demonstrated dramatically higher βENaC expression on alveolar luminal surfaces in the Nedd4-2 −/− lung compared with wild type ( Fig. 3c ). E18.5 kidneys from Nedd4-2 −/− animals also showed a clear increase of βENaC in the membranes of collecting ducts compared with wild-type littermates ( Fig. 3c ). Together, these results are consistent with a role for Nedd4-2 in ENaC regulation. 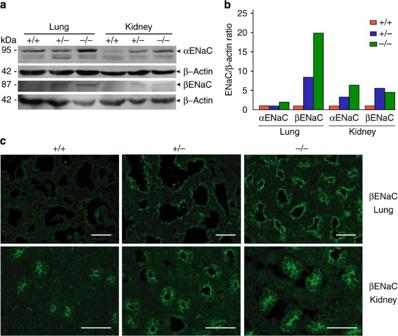Figure 3: Increased ENaC expression inNedd4-2−/−mice. (a) α and βENaC expression in E18.5 lung and kidney. (b) Quantification of ENaC expression from (a) normalized to β-actin and relative to wild type. (c) βENaC expression (green) in E18.5 lung and kidney. Scale bars, 50 μm. Figure 3: Increased ENaC expression in Nedd4-2 −/− mice. ( a ) α and βENaC expression in E18.5 lung and kidney. ( b ) Quantification of ENaC expression from ( a ) normalized to β-actin and relative to wild type. ( c ) βENaC expression (green) in E18.5 lung and kidney. Scale bars, 50 μm. Full size image As ENaC is also expressed in the skin and has been implicated in epidermal differentiation [24] , [25] , we assessed whether loss of Nedd4-2 affects ENaC expression and skin differentiation. Skin sections from Nedd4-2 wild-type, Nedd4-2 +/− and Nedd4-2 −/− mice were analysed for expression of various skin differentiation markers. There were no obvious differences observed in skin using markers of epidermal differentiation from embryos (E16.5), neonates (P1) or survivors at P19 ( Supplementary Fig. S4 ). Furthermore, there were no obvious differences in βENaC expression in the skin of P1 and P19 wild-type and Nedd4-2 −/− animals ( Supplementary Fig. S5 ). These results suggest that Nedd4-2 does not have a major role in ENaC regulation in the epidermis and that epidermal differentiation in skin occurs normally in the absence of Nedd4-2. Increased ENaC function in Nedd4-2 −/− mice To determine whether the increased ENaC expression observed at the alveolar surface of E18.5 Nedd4-2 −/− lungs correlates with increased amiloride-sensitive sodium current due to ENaC, whole-cell patch clamp recording was performed on alveolar type II lung cells ( Fig. 4a ). The presence of Na + current was initially assessed by replacing 140 mM extracellular Na + with equimolar amounts of the impermeant cation N -methyl- D -glucamine ( Fig. 4b ). If Na + current was present, 50 μM amiloride was applied to the bath solution to ascertain if the current was mediated by ENaC ( Fig. 4b ). The I–V current/voltage plots of ENaC currents in Nedd4-2 +/+ and Nedd4-2 −/− cells obtained by subtracting current traces recorded before and after the application of amiloride showed strong inward rectification and reversal potential of approximately +50 mV, which is characteristic of a Na + -selective channel ( Fig. 4c ). The average amplitude of amiloride-sensitive Na + current measured at −100 mV in lung cells isolated from Nedd4-2 +/+ animals was −2.2±0.4 pA/pF ( n =19), whereas current measured in Nedd4-2 −/− cells had a significantly greater amplitude of −15.1±3.2 pA/pF ( n =8; P <0.0001; Fig. 4d ). These data indicate that the loss of Nedd4-2 is strongly correlated with increased ENaC current in alveolar type II cells. 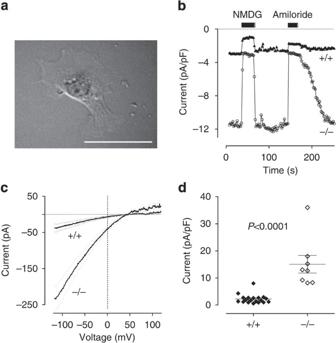Figure 4: ENaC-mediated current in lung cells. (a) A typical isolated epithelial lung cell producing ENaC current. Scale bar, 20 μm. (b) The effects of Na+replacement with an impermeant cation (N-methyl-D-glucamine, NMDG) and the application of amiloride on the whole-cell membrane currents of lung cells isolated from wild-type andNedd4-2−/−mice. NaCl (140 mM) was replaced with 140 mM NMDGCl in the external solution and 50 μM amiloride was applied into the bath. Each point represents amplitude of the current at −100 mV measured from responses to the voltage ramps ranging from −120 to 120 mV and applied every 2 s. Representative cells are shown. (c) Averaged I–V plots of amiloride-sensitive currents in wild-type (n=19) andNedd4-2−/−(n=8) lung cells. Black lines represent averaged current traces obtained in response to voltage ramps ranging from −120 to 120 mV. Dashed grey lines represent s.e.m. (d) The amplitudes of the amiloride-sensitive current measured at −100 mV in wild-type (filled symbols,n=19) andNedd4-2−/−(clear symbols,n=8) cells. Horizontal lines represent the mean±s.e.m.P<0.0001 was determined by unpaired two-tailt-test. Figure 4: ENaC-mediated current in lung cells. ( a ) A typical isolated epithelial lung cell producing ENaC current. Scale bar, 20 μm. ( b ) The effects of Na + replacement with an impermeant cation ( N -methyl- D -glucamine, NMDG) and the application of amiloride on the whole-cell membrane currents of lung cells isolated from wild-type and Nedd4-2 −/− mice. NaCl (140 mM) was replaced with 140 mM NMDGCl in the external solution and 50 μM amiloride was applied into the bath. Each point represents amplitude of the current at −100 mV measured from responses to the voltage ramps ranging from −120 to 120 mV and applied every 2 s. Representative cells are shown. ( c ) Averaged I–V plots of amiloride-sensitive currents in wild-type ( n =19) and Nedd4-2 −/− ( n =8) lung cells. Black lines represent averaged current traces obtained in response to voltage ramps ranging from −120 to 120 mV. Dashed grey lines represent s.e.m. ( d ) The amplitudes of the amiloride-sensitive current measured at −100 mV in wild-type (filled symbols, n =19) and Nedd4-2 −/− (clear symbols, n =8) cells. Horizontal lines represent the mean±s.e.m. P <0.0001 was determined by unpaired two-tail t -test. Full size image Nedd4-2 +/− mice show a trend towards hypertension As discussed previously, Nedd4-2 heterozygous mice express intermediate levels of Nedd4-2 protein, leading to intermediate levels of α and βENaC total protein in kidneys and an intermediate level of βENaC expression in the collecting duct epithelia compared with wild type and Nedd4-2 −/− ( Fig. 3 ). As ENaC in the kidney is tightly regulated, a small increase in ENaC expression may result in measurable changes in blood pressure. Nedd4-2 +/− mice showed no overt phenotype or gross abnormalities and have a lifespan similar to wild-type littermates. On a normal salt diet (0.3% Na + ) Nedd4-2 +/− mice had an elevated baseline blood pressure (109.4±3.1 mm Hg, n =8, P =0.085) compared with wild type (87.1±8.4 mm Hg, n =4). However, after 14 days on a high salt (3.1%) diet, there was no statistically significant difference between the blood pressure of wild-type (85.2±19.4 mm Hg, n =4) and Nedd4-2 +/− mice (92.5±15.1 mm Hg, n =8, P =0.484). We also performed electrocardiography on adult wild-type and Nedd4-2 +/− mice. There were no significant differences observed in any parameters tested ( Supplementary Table S1 ). From these data we conclude that although the loss of one copy of Nedd4-2 may predispose animals to hypertension, their heart and vascular functions appear normal. Inflammatory lung disease in Nedd4-2 −/− survivors As stated previously a small number ( ∼ 4.2%) of Nedd4-2 −/− animals survive up to a maximum of 22 days of age. We analysed the possible cause of lethality in these mice. The lung architecture of surviving Nedd4-2 −/− mice was the same as wild type at P10 ( Fig. 5a,b ); however, the increased level of βENaC expression in the lung compared with wild-type littermates persisted at P21 ( Fig. 5c,d ), indicating this phenotype is chronic from birth. Lung sections from a Nedd4-2 −/− animal that died at P21 demonstrated extensive fibrosis in the alveolar spaces compared with wild-type littermates ( Fig. 5e–i ). We also observed significant cellular infiltrate in lung tissue and air spaces of Nedd4-2 −/− survivors examined, and the amount of infiltrate varied between animals. At higher magnification different types of inflammatory cells such as macrophages and neutrophils were clearly visible in alveolar spaces ( Fig. 5g ). 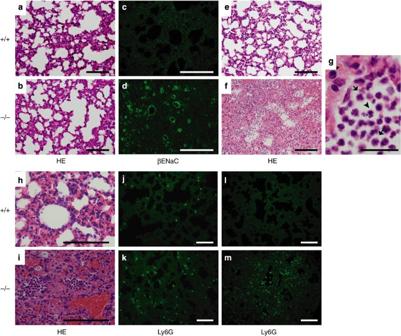Figure 5: SurvivingNedd4-2−/−mice develop lung inflammation. Lung sections ofNedd4-2+/+andNedd4-2−/−mice. (a,b) Haematoxylin and eosin (HE) stained P10 lung. (c,d) βENaC expression in P21 lung sections. (e,f) HE stained P21 lung. (g) Enlarged view of a section inf. Arrowhead indicates a macrophage, arrows indicate neutrophils. (h,i) HE stained P21 lung at higher magnification. (j,k) Ly6G staining neutrophils in P14 lung. (l,m) Ly6G staining in P19 lung. Scale bars represent 100 μm except ingwhere it represents 20 μM. Figure 5: Surviving Nedd4-2 −/− mice develop lung inflammation. Lung sections of Nedd4-2 +/+ and Nedd4-2 −/− mice. ( a , b ) Haematoxylin and eosin (HE) stained P10 lung. ( c , d ) βENaC expression in P21 lung sections. ( e , f ) HE stained P21 lung. ( g ) Enlarged view of a section in f . Arrowhead indicates a macrophage, arrows indicate neutrophils. ( h , i ) HE stained P21 lung at higher magnification. ( j , k ) Ly6G staining neutrophils in P14 lung. ( l , m ) Ly6G staining in P19 lung. Scale bars represent 100 μm except in g where it represents 20 μ M . Full size image To confirm the presence of inflammatory cells, immunofluorescence staining was performed on lung sections from the survivors with a neutrophil-specific antibody. Lungs from Nedd4-2 −/− survivors showed an increased number of neutrophils compared with wild-type as early as P14, and this was further increased in the Nedd4-2 −/− lung at P19 ( Fig. 5j–m ). Bronchoalveolar lavage (BAL) was performed on Nedd4-2 −/− survivors and wild-type mice to measure neutrophil- and macrophage-specific chemokines (keratinocyte-derived chemokine (KC) and macrophage inflammatory protein-2 (MIP-2), respectively), and KC levels were considerably higher in Nedd4-2 −/− BAL fluid compared with wild type ( Table 2 ). Table 2 Chemokine and cytokine levels in alveolar lung fluid of P16 Nedd4-2 −/− mice. Full size table Nedd4-2 has been implicated in regulating the processing and levels of surfactant protein-C (SP-C), a pulmonary surfactant protein secreted by alveolar type II cells [26] , [27] . However, we found that SP-C staining was similar in lung sections from both Nedd4-2 −/− and Nedd4-2 +/+ littermates ( Fig. 6a,b ). Furthermore, mucin levels in the lung of Nedd4-2 −/− and Nedd4-2 +/+ littermates were comparable ( Fig. 6c,d ) as were mucous levels ( Fig. 6e,f ). No bacterial infection was observed in either lung or spleen homogenates of Nedd4-2 −/− survivors at P14, and there were a lack of CD4 + T cells in Nedd4-2 +/+ and Nedd4-2 −/− lungs, consistent with sterile inflammation. Indeed, ultrastructural examination of a P19 lung by transmission electron microscopy (TEM) commonly identified pyknotic nuclei in Nedd4-2 −/− survivor lungs, indicating the occurrence of necrosis in the alveolar epithelium ( Fig. 6g,h ). 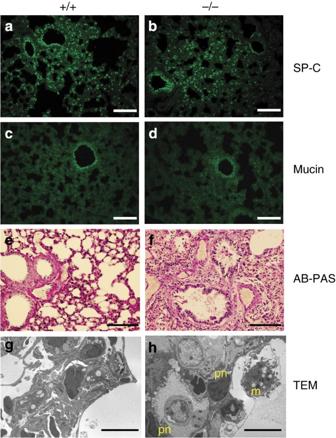Figure 6: Lung phenotype of survivingNedd4-2−/−mice is not due to altered surfactants or mucous. (a,b) Surfactant Protein-C expression in P14 lung. (c,d) Mucin expression in P14 lung. (e,f) Alcian-blue/periodic acid-Schiff (AB-PAS) staining mucopolysaccharides in P21 lung. (g,h) TEM of P19 lung, with pyknotic nuclei (pn) and a macrophage (m) indicated. Scale bars represent 100 μm except ing,hwhere it represents 10 μM. Figure 6: Lung phenotype of surviving Nedd4-2 −/− mice is not due to altered surfactants or mucous. ( a , b ) Surfactant Protein-C expression in P14 lung. ( c , d ) Mucin expression in P14 lung. ( e , f ) Alcian-blue/periodic acid-Schiff (AB-PAS) staining mucopolysaccharides in P21 lung. ( g , h ) TEM of P19 lung, with pyknotic nuclei (pn) and a macrophage (m) indicated. Scale bars represent 100 μm except in g , h where it represents 10 μ M . Full size image Despite extensive in vitro evidence that suggests Nedd4-2 regulates several membrane proteins [4] , the physiological role of Nedd4-2 remains poorly understood. The present study demonstrates that Nedd4-2 is a key in vivo regulator of ENaC function in the lung and is critical for animal survival. The absence of Nedd4-2 leads to an increase in ENaC expression and sodium conductance in lung epithelial cells, which has lethal physiological consequences. The most striking feature of the Nedd4-2 −/− mice is their perinatal lethality. Over 95% of the Nedd4-2 −/− mice die soon after birth because of respiratory distress, whereas the 4.2% of Nedd4-2 −/− mice that survive develop significant fibrosis and inflammation of the lung leading to their death by day 22. One of the key targets of Nedd4-2 is ENaC, which is essential for electrolyte balance and for regulating respiratory epithelial fluid [11] . The Nedd4-2 −/− mice we generated in this study show a significant increase of ENaC expression and activity in the lung epithelium. ENaC expression begins a few days before birth. We suggest that the increased pulmonary sodium absorption due to the observed increased ENaC activity at E18.5 results in premature alveolar fluid clearance, as also evident from the decreased wet/dry ratios in lungs at this stage. This in turn presumably leads to the observed structural collapse of the alveoli at E18.5 in Nedd4-2 −/− mice, resulting in perinatal death due to respiratory distress. Increased alveolar fluid clearance due to ENaC hyperactivity is also observed in β-Liddle mice, which have a mutation introduced into βENaC that prevents its downregulation by Nedd4-2, whereas maintaining wild-type levels of both α and γENaC [28] , [29] , [30] . Thus, although we cannot rule out that the absence of Nedd4-2 affects other channels, it seems very likely that the correct regulation of ENaC by Nedd4-2 in vivo is critical for animal survival. Mice lacking Nedd4-2 present a somewhat similar phenotype to βENaC overexpressing mice, in which the increased βENaC levels leads to a decreased amount of luminal fluid in the lungs and reduced mucous transport, neutrophillic inflammation and poor bacterial clearance [14] , [31] . Recent studies have shown that the overexpression of βENaC in transgenic mouse lungs results in airway surface dehydration that causes chronic lung inflammation with a high neonatal pulmonary mortality, sterile inflammation due to epithelial necrosis and chronic bronchitis in adult survivors [32] . The observed airway inflammation included macrophage activation, eosinophil and neutrophil recruitment, and elevated KC and tumor necrosis factor-α chemokine levels [31] . Given that Nedd4-2 −/− survivor mice similarly display epithelial necrosis, lung infiltration by neutrophils and macrophages, and elevated KC chemokine levels, this suggests that overexpression of ENaC in the lung of Nedd4-2 −/− mice is the principal cause of the observed phenotypes. Surviving Nedd4-2 −/− mice show wild-type levels of SP-C proprotein, a critical regulator of alveolar surface tension in the lungs, which is consistent with the normal lung architecture observed in these animals. However, increased ENaC expression is likely to trigger the lethal inflammation of the lung in Nedd4-2 −/− survivor mice due to sodium hyperabsorption, and the observed epithelial necrosis constitutes a mechanism to initiate inflammation in the absence of bacterial infection. Indeed, a recent report described a conditional Nedd4-2 knockout in the lung that resulted in a cystic fibrosis-type lung phenotype, somewhat similar to the observations reported in this manuscript [33] . An independent Nedd4-2 knockout line generated previously by Shi and co-workers (Yang mice) has been reported as viable and generally healthy except showing a mild salt-sensitive hypertension and cardiac hypertrophy [22] . Surprisingly, these Nedd4-2 knockout mice displayed no lung phenotype. This phenotype is similar to our Nedd4-2 heterozygous mice, which showed a slight tendency towards elevated blood pressure compared with wild-type and no lung phenotype. We were unable to perform blood pressure measurements on our Nedd4-2 −/− mice as most die at birth, and survivors only live to a maximum age of 22 days. The Yang mice have a much milder phenotype than would be expected if Nedd4-2 was a major regulator of ENaC. Altering the expression of even a single subunit of ENaC, such as in the βENaC overexpressing transgenic mice [14] , [32] , results in a more extreme phenotype than the Yang Nedd4-2 knockout mice [22] . In addition single-nucleotide polymorphisms in human NEDD4-2 ( NEDD4L ) have been linked to hypertension [34] , so a complete Nedd4-2 knockout would be expected to show more than a mild hypertensive phenotype. By analysing the Yang mice, we detected Nedd4-2 mRNA and protein bands indicating an incomplete knockout, probably due to a readthrough transcript(s) and alternative splicing ( Supplementary Fig. S1 ). Our Nedd4-2 −/− mice on the other hand showed no evidence of Nedd4-2 mRNA or protein expression ( Supplementary Fig. S1 ). It is possible that the mixed genetic background of the Yang knockout mice also contributes to the milder phenotype of these mice compared with the Nedd4-2 −/− mice described in this study. In preliminary studies, we noticed that when our Nedd4-2 −/− mice were crossed into a SV129J background to generate a mixed SV129J/C57Bl6 genetic background, the perinatal lethality of our Nedd4-2 −/− mice was significantly rescued, with mice surviving up to 25 days before dying of lung inflammation ( Supplementary Fig. S6 ). This suggests that both a mixed genetic background and hypomorphic nature contribute to the lack of phenotype in the Yang knockout mice. Our data clearly demonstrate that Nedd4-2 is a critical regulator of ENaC function in the lung. Our Nedd4-2 −/− mice show increased ENaC expression in the lung and kidney. This increased ENaC expression in the embryonic lung appears to result in perinatal lethality due to an inability to inflate the lungs and respiratory failure. The few Nedd4-2 −/− animals that survive birth have persistent ENaC overexpression and develop lethal inflammation of the lung within a few weeks. Nedd4-2 has been implicated in the regulation of a number of other proteins [4] . However, many of these targets, such as the voltage-gated sodium and potassium channels, dopamine and glutamate transporters and Trk are unlikely to contribute to the lung phenotype. Furthermore, we have shown here that the loss of Nedd4-2 does not affect animal development and the Nedd4-2 −/− animals do not show other overt abnormalities except for the pulmonary phenotype. This suggests that, unlike Nedd4 that is essential for growth and development [5] , Nedd4-2 is not a critical regulator of proteins and pathways involved in animal development. Although it is possible that regulation of additional proteins contribute to the inflammatory lung phenotype in surviving Nedd4-2 −/− animals, our data clearly indicate that Nedd4-2 is essential for the regulation of ENaC and for animal survival. Generation of Nedd4-2 knockout mice The Nedd4-2 disruption vector consists of a 5,010 bp 5′ homology arm that incorporates Nedd4-2 exons 13, 14 and part of 15, a loxP site inserted in a forward orientation within exon 15 that contains a stop codon, a Pgk promoter driven neomycin phosphotransferase resistance gene followed by another loxP site and then the 6,310 bp 3′ homology arm that incorporates part of exon 16 and exon 17 of Nedd4-2 in the targeting vector backbone pLOz. The targeting construct was linearized and electroporated into Bruce4 C57BL/6 ES cells [23] . G418-resistant ES colonies were analysed for correct integration and confirmed by Southern blotting. Chimeras were generated from ES clones by blastocyte injection, backcrossed to C57BL/6J and offspring analysed by Southern blotting. Chimeric mice containing the disruption vector were crossed to Cre deleter mice (Ozgene) to generate founding Nedd4-2 knockout mice. Animals were maintained in the SA Pathology animal facility. All animal procedures were approved by the SA Pathology Animal Ethics Committee and experiments were performed according to the guidelines provided by the National Health and Medical Research Council. Morphology Collected embryos were washed in PBS, dissected and organs placed in Histochoice MB fixative (Electron Microscopy Sciences) overnight at 4 °C. Organs were immersed in 30% sucrose for 24 h at 4 °C, embedded in Tissue-Tek® Optimal Cutting Temperature (OCT) compound and stored at −70 °C. Ten-micrometre-thick sections were stained with haematoxylin and eosin or Alcian-blue/periodic acid-Schiff. For skin analysis, embryos were fixed in 4% paraformaldehyde for at least 24 h, embedded in paraffin wax and cut. After wax removal (Histolemon) sections were rehydrated in alcohol/distilled water and microwave-assisted antigen retrieval was performed in 0.01 M sodium citrate (pH 6). Sections were incubated in 0.1 M NaBH 4 overnight at 4 °C to reduce tissue auto-fluorescence. Lung samples for TEM were fixed in TEM fixative (4% paraformaldehyde/1.25% glutaraldehyde in PBS, and 4% sucrose, pH 7.2) for several days and washed in PBS. Processing was performed in a PELCO BioWave microwave oven (PELCO). Samples were postfixed in 1% aqueous osmium tetroxide, dehydrated in a graded series of acetones, and infiltrated with Procure/Araldite epoxy resin. Blocks were polymerized overnight at 70 °C. Sections were cut on a Leica UltraCut S Ultramicrotome (Leica) using a diamond knife and stained with uranyl acetate and lead citrate. Caesarian recovery and hydrostatic lung test Embryos were colleced at E18.5, placed on a 37 °C heat pad and observed. Embryos were decapitated after 60 min observation, and lungs with trachea, heart and thymus still attached were placed into water and observed for floatation. The lungs were then cut into 12–20 small pieces and again immersed in water and flotation recorded. Lung wet/dry measurements Lungs were isolated from pups collected at E17.5 or E18.5, blotted on filter paper and weighed to obtain wet lung weight. The lungs were then incubated overnight at 85 °C and weighed to obtain dry lung weight. Blood pressure measurements Wild-type and Nedd4-2 +/− littermates aged between 20–24 weeks were kept on a normal salt diet (0.36% sodium) and acclimatized to the blood pressure procedure 7–10 days before baseline measurements. Blood pressure was measured in the afternoon using the volume pressure sensor tail cuff method, using a CODA6 non-invasive blood pressure apparatus (Kent Scientific). Mice were switched to a high salt diet (3.1% sodium, Specialty Feeds), and blood pressure measurements taken at 7 and 14 days after the start of high salt dietary regime. The CODA6 acquisition system was used to record diastolic, systolic and mean blood pressure, tail blood volume and flow. Lung cell preparation and patch clamping E18.5 lungs were perfused with 1.4 U ml −1 heparin solution and digested with 20 U of Elastase pancreatic Solution Type I from porcine pancreas (Sigma). Dissociated lung pieces were panned over bovine IgG-coated plastic dishes for 90 min at 37 °C before plating on acid-washed coverslips in DMEM media containing 10% FCS. Whole-cell patch clamping was performed as previously described [35] . Antibody production and purification Polyclonal rabbit anti-βENaC serum was generated using the recombinant peptide sequence (CQPLDTMESDSEVEAI) from mouse βENaC as the immunogen. A polyclonal rabbit anti-αENaC serum was generated using the peptide sequence (YRYTEIKEDLEELDRITEQT) from mouse αENaC. Serum was affinity purified against the αENaC peptide coupled to cyanogen bromide-activated Sepharose. Bound proteins were eluted into Tris-HCl (pH 8.6) with 100 mM glycine (pH 2.5) and dialysed against PBS. Anti-ENaC sera were preadsorbed overnight at 4 °C with the relevant peptide antigen, and used as a control in immunoblotting and immunohistochemistry to test the specificity of antibodies in detecting ENaC. Immunoblot analysis Tissues collected from E18.5 mice were placed into ice-cold buffer (150 mM NaCl, 5 mM EDTA, 50 mM Tris-HCl pH7.4, 0.1% SDS, 1% NP40, 0.5% NaDOC+Roche Complete Protease Inhibitors (Roche)) on ice. Tissues were homogenized, incubated at 4 °C on a shaking platform for 30 min, centrifuged at 16,000 r.p.m. for 5 min. Supernatant proteins (100 μg) were resolved in 10% SDS–polyacrylamide gel electrophoresis then transferred to PVDF membrane (Perkin-Elmer) and membranes were blocked in 5% skim milk in PBS-T. Primary antibodies added were either mouse monoclonal anti-Nedd4 antibody (BD Transduction), rabbit polyclonal anti-Nedd4-2 antibody [36] , mouse β-actin (Sigma-Aldrich), anti-βENaC serum or anti-αENaC affinity purified antibody. Secondary antibodies were added at 1:2,000: either goat anti-rabbit conjugated alkaline phosphatase (Southern Biotech) or goat anti-mouse conjugated alkaline phosphatase (Millipore) and visualized with ECF substrate (Amersham) on a Typhoon 9410 (Molecular Dynamics). Serum depleted of specific antibodies by preabsorbtion with peptide antigen was used as control where appropriate. Northern blot analysis Total tissue RNA was extracted using Trizol reagent (Invitrogen) as per manufacturer's protocol. Thirty micrograms of RNA was electrophoresed on formaldehyde gel, transferred to Hybond N membrane (Amersham) and hybridized to a 32 P-labelled full-length Nedd4-2 cDNA probe using standard protocols. Membranes were washed and phosphoimaged using a Typhoon 9410 (Molecular Dynamics). Microscopy Confocal images were captured using a Bio-Rad Radiance 2100 confocal microscope (Bio-Rad) equipped with Argon ion 488 nm, Green HeNe 543 nm and Red Diode 637 nm lasers, imaged in water at 20 °C, and captured using LAsersharp2000 software and EZ-C1 software. The objectives used were ×20 UAPOW (NA=0.70), ×40 UPLAPO (NA=1.15) and ×60 UPLAPO with NA=1.4 water. Light images were captured with an Olympus BX51 microscope (Olympus), Olympus DP70 camera (Olympus), imaged at room temperature using Olysia Bioreport software. The objectives used were ×10 UPlanApo (NA=0.4) ×20 UPlanApo (NA=0.7) and ×40 UPlanApo (NA=0.85). TEM images were captured on a Philips CM100 Transmission Electron Microscope (Philips) and imaged using iTEM 5.0 (Build 1131) software. Immunofluorescence staining For immunofluorescent staining of lung, kidney and skin sections the following primary antibodies were used: anti-βENaC, Ly6G (BD Pharmingen), Surfactant Protein C (Abcam), anti-Mucin 5AC (Abcam), anti-mouse monoclonal CD4 (BD Pharmingen), monoclonal anti-p63 Ab4 (Neomarkers), polyclonal anti-MK14 (Covance), polyclonal anti-MK10 (Covance), polyclonal anti-loricrin (Covance) and polyclonal anti-loricrin (Covance). Sections were incubated for 1 h at room temperature with either biotinylated sheep anti-rabbit IgG (Rockland), biotinylated goat anti-rat IgG (Jackson Immunoresearch) or biotin-conjugated sheep anti-mouse IgG (Amersham), washed and incubated with streptavidin-conjugated AlexaFluor 488 (Molecular Probes) diluted 1:250 in PBS for 30 min at room temperature. The secondary antibody for CD4 staining was goat anti-rat FITC 1:250 (Zymed). Sections were mounted with Antifade. Serum depleted of specific antibodies by preadsorbtion with peptide antigen was used as control where appropriate. Bronchoalveolar lavage and chemokine and cytokine measurement Nedd4-2 −/− survivors and wild-type littermates were euthanized and dissected to expose the trachea and thoracic cavity. A 26-gauge needle was inserted through the trachea and lungs were lavaged with 500 μl of ice-cold PBS. BAL fluid was centrifuged at 300 g and supernatants collected and measured for MIP-2, KC, interleukin-1α and interleukin-1β using DuoSet ELISA kits (R&D systems). Measurement of bacterial burden Lung tissue and spleen from Nedd4-2 −/− survivors and wild-type littermates were weighed, homogenized in Luria broth (LB) and centrifuged at 400 g for 5 min. Supernatants were collected and used neat or diluted 1:10 or 1:100 in LB before plating 50 μl onto LB agar and incubating overnight at 37 °C. Statistical analysis Unless stated otherwise, statistical analyses were performed using unpaired t -test assuming equal variance, with statistical significance determined as being P <0.05. χ 2 analysis was performed using the online calculation chi-square tool at http://www.quantpsy.org . How to cite this article: Boase, N. A. et al . Respiratory distress and perinatal lethality in Nedd4-2-deficient mice. Nat. Commun. 2:287 doi: 10.1038/ncomms1284 (2011).